60S ribosome biogenesis requires rotation of the 5S ribonucleoprotein particle During eukaryotic ribosome biogenesis, nascent ribosomal RNA (rRNA) forms pre-ribosomal particles containing ribosomal proteins and assembly factors. Subsequently, these immature rRNAs are processed and remodelled. Little is known about the premature assembly states of rRNAs and their structural rearrangement during ribosome biogenesis. Using cryo-EM we characterize a pre-60S particle, where the 5S rRNA and its associated ribosomal proteins L18 and L5 (5S ribonucleoprotein (RNP)) are rotated by almost 180° when compared with the mature subunit. Consequently, neighbouring 25S rRNA helices that protrude from the base of the central protuberance are deformed. This altered topology is stabilized by nearby assembly factors (Rsa4 and Nog1), which were identified by fitting their three-dimensional structures into the cryo-EM density. We suggest that the 5S RNP performs a semicircular movement during 60S biogenesis to adopt its final position, fulfilling a chaperone-like function in guiding the flanking 25S rRNA helices of the central protuberance to their final topology. During eukaryotic ribosome formation, a large number of biogenesis factors catalyse the intricate assembly of ribosomal RNA (rRNA) and ribosomal proteins into the two ribosomal subunits [1] , [2] , [3] , [4] . Newly synthesized rRNA folds co-transcriptionally and recruits r-proteins and assembly factors to form the early pre-ribosomal particles, which gradually evolve through a series of intermediates into mature ribosomes [5] , [6] , [7] , [8] . Along this pathway, the immature rRNA requires extensive modification, processing and structural remodelling [1] . Three of these rRNA molecules—18S rRNA of the small (40S) ribosomal subunit as well as 5.8S and 25S/human 28S rRNAs of the large (60S) ribosomal subunit—are initially transcribed in the nucleolus by RNA polymerase I as a larger rRNA precursor (35S rRNA in yeast; 45S rRNA in human). In contrast, 5S rRNA is transcribed separately by RNA polymerase III, and its precursor matures to the 5S rRNA independently from the pre-35S RNA processing pathway [9] , [10] . Subsequently, 5S rRNA recruits two r-proteins, L5 and L18 (previously called Rpl11 and Rpl5 in yeast, respectively), to form the 5S ribonucleoprotein (RNP) particle, which becomes incorporated en bloc into the evolving pre-60S subunit [11] , [12] , [13] . In the mature 80S ribosome, the 5S rRNA is located within the central protuberance of the 60S subunit, where it is involved in intersubunit interactions, mediated by a number of protein–RNA and RNA–RNA contacts [14] , [15] . A multitude of transiently interacting ribosome assembly factors participate in a complicated cascade of assembly and maturation reactions, which take place during 40S and 60S subunit formation [16] . The earliest pre-ribosomal biogenesis intermediates are located in the nucleolus, which subsequently go through a series of nucleolar–nucleoplasmic transition states to develop into medium and late-stage nucleoplasmic particles. Eventually, these particles gain nuclear export competence and are transported to the cytoplasm, where final maturation takes place [17] . Despite the advances in our compositional understanding, only little structural data is available for pre-60S particles, and structural information on the ribosomal interaction of assembly factors has mostly been gained using reconstitution with mature subunits [18] , [19] , [20] , [21] . We recently solved the first cryo-EM structure of a native pre-60S particle in association with the assembly factor Arx1 at 12 Å resolution [22] . This EM map revealed structural differences between the pre-60S particle and mature 60S subunit demonstrating the need of comprehensive structural investigations of native pre-ribosomal particles. Here, we present the first sub-nanometre cryo-EM structure of a eukaryotic 60S ribosomal subunit assembly intermediate, and position several biogenesis factors—Rlp7, Rlp24, Mrt4, Nog1 and Rsa4—within this structure. Unexpectedly, the preassembled 5S RNP, consisting of the 5S rRNA and ribosomal proteins L18 and L5, is found in a radically different topology when compared with the native 60S subunit. Thus, our results give insight into the folding and assembly pathway of the large ribosomal subunit rRNA. Cryo-EM structure of a eukaryotic pre-60S ribosomal subunit To gain the desired in-depth structural insight into the architecture of the nascent 60S subunit, we have now determined the structure of an Arx1 particle [23] , affinity-purified via the bait protein Alb1 (ref. 22) [22] , by cryo-EM at sub-nanometre (8.7 Å) resolution ( Fig. 1 ; Supplementary Fig. 1 ). Importantly, at this resolution all helical rRNA structures as well as most secondary structures of proteins can be assigned, allowing for the first time to generate a molecular model of a nascent pre-60S subunit ( Supplementary Fig. 2 ). 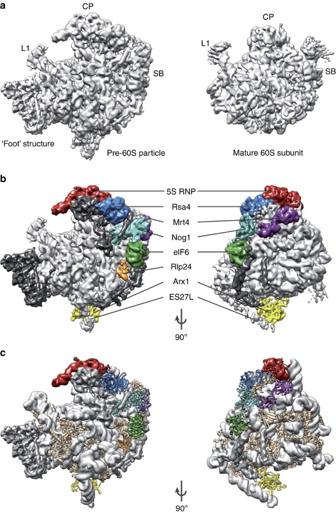Figure 1: Cryo-EM structure and model of the Arx1 pre-60S particle. (a) The cryo-EM reconstruction of theS. cerevisiaeArx1 particle at 8.7 Å resolution (left) and the mature 60S subunit (right, isolated from yeast RNC-Ssh1 (ref. 49)49). L1: L1-stalk; CP: central protuberance; SB: stalk base. (b) Segmentation of the cryo-EM reconstruction highlighting the 5S RNP (red), Rsa4 (blue), Mrt4 (purple), eIF6 (green) and Arx1 (yellow) as well as the respective N-terminal domains of Nog1 (cyan) and Rlp24 (orange). The pre-60S subunit and non-assigned density are depicted in light and dark grey, respectively. ES27L: expansion segment 27 of the large subunit rRNA. (c) Model for the Arx1 particle. rRNA is represented as artificial density (at 8 Å resolution in light grey) and proteins as ribbons. The experimental density is shown in dark grey for regions of the reconstruction that are not represented by the model. Ribosomal proteins are depicted in light brown, other colours as in (b). Figure 1: Cryo-EM structure and model of the Arx1 pre-60S particle. ( a ) The cryo-EM reconstruction of the S. cerevisiae Arx1 particle at 8.7 Å resolution (left) and the mature 60S subunit (right, isolated from yeast RNC-Ssh1 (ref. 49) [49] ). L1: L1-stalk; CP: central protuberance; SB: stalk base. ( b ) Segmentation of the cryo-EM reconstruction highlighting the 5S RNP (red), Rsa4 (blue), Mrt4 (purple), eIF6 (green) and Arx1 (yellow) as well as the respective N-terminal domains of Nog1 (cyan) and Rlp24 (orange). The pre-60S subunit and non-assigned density are depicted in light and dark grey, respectively. ES27L: expansion segment 27 of the large subunit rRNA. ( c ) Model for the Arx1 particle. rRNA is represented as artificial density (at 8 Å resolution in light grey) and proteins as ribbons. The experimental density is shown in dark grey for regions of the reconstruction that are not represented by the model. Ribosomal proteins are depicted in light brown, other colours as in ( b ). Full size image Compared with the mature 60S subunit, the reconstruction of the Arx1 particle displays additional densities and, as only revealed at the current sub-nanometre resolution, a completely rearranged central protuberance ( Fig. 1 ; Supplementary Figs 3 and 4 ). The additional densities cluster at the functional sites of the 60S subunit, whereas the solvent side of the pre-60S subunit is very similar to its mature state, and is nearly devoid of additional density [22] . Notably, with the new cryo-EM map at 8.7 Å resolution, we could trace the fully assembled 5S RNP including its 5S rRNA and bound r-proteins L5 and L18 on top of the pre-60S particle, but in a radically different orientation (see below). This unexpected finding is consistent with the incorporation of a preformed 5S RNP into the pre-60S subunit [11] . Moreover, the higher resolution cryo-EM map allowed us to assign, in addition to the previously identified biogenesis factors Arx1 (refs 19 , 22 ) and eIF6 (refs 18 , 20 ), the precise locations of Rlp7, Rlp24, Mrt4, Nog1 and Rsa4 on the Arx1 particle. Initially, the Arx1 particle was identified as an export-competent particle with bound export factors Nmd3 and Mex67-Mtr2 that follows the Rix1–Rea1 remodelling step [16] , [22] . Therefore, the identification of Rsa4 within our current cryo-EM map of the Arx1 particle was unexpected and suggested that this pre-60S intermediate did not yet undergo the Rix1/Rea1-dependent remodelling step, which is known to cause the dissociation of Rsa4 (ref. 24) [24] . To clarify this apparent contradiction, we further separated our Arx1 particle preparation according to the presence or absence of Rsa4 by an additional affinity chromatography step using Flag-tagged Rsa4. Western blot analysis revealed that this segregated the particles into two distinct populations: as expected, the Rsa4-free particles indeed contained the previously described export factors, whereas the Rsa4-bound fraction carried a different set of assembly factors lacking the export factors Nmd3 and Mex67 ( Supplementary Fig. 5 ). Thus, we conclude that a pool of early Arx1 particles exists, which is ‘upstream’ of the Rix1 particle and apparently corresponds to the distinct cryo-EM structure described in the previous [22] and present study. However, following the Rix1–Rea1 remodelling step and removal of Rsa4, the Arx1 particle progresses towards the mature 60S subunit by recruiting the nuclear export factors (for example, Nmd3, Crm1 and Mex67) and transport to the cytoplasm (for model see Supplementary Fig. 5 ). We checked for the presence of the large subunit r-proteins in our 60S assembly intermediate ( Supplementary Table 1 ; Supplementary Fig. 6 ). Densities were absent for L29e, L44e and the P1 and P2 proteins indicating that these proteins have not yet assembled into the pre-particle. In addition, the binding sites of L16 and L41e are not used by these proteins yet, but are instead occupied by rRNA helix 89 and helix 71, respectively. Also L40e appears to be absent, which is in agreement with a previous study showing that L40e, like L16 (refs 25 , 26 ), is assembled into the maturing 60S subunit only in the cytoplasm [27] . Next, we attempted to identify the positions of additional assembly factors that we found to be enriched in the Arx1 particle according to mass spectrometry or western blot analysis ( Supplementary Fig. 5 ). 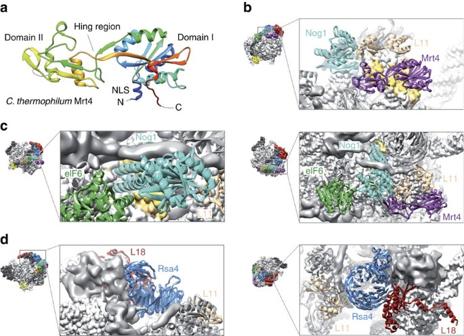Figure 2: Ribosome assembly factors and their binding sites on the pre-60S subunit. (a) Crystal structure ofChaetomium thermophilumMrt4 at 1.8 Å resolution. (b) Nog1 extends its tripod-like N-terminal domain into the distorted A- and P-sites contacting the 25S rRNA near helices 42, 89 and 90. Its GTPase domain binds to the tip of the Sarcin–Ricin loop in close proximity to eIF6, Mrt4 and L11. (c) Rsa4 binds between the 5S RNP and the stalk base in close proximity to L18 and L11. (d) Mrt4 binds to the stalk base close to Nog1 and L11. Its binding mode resembles that of P0. Protein models and crystal structures are depicted as ribbons, rRNA models (white) are depicted as density at 3.5 Å resolution, and non-interpreted density is shown in dark grey. Contact regions between ribosome assembly factors and the 25S rRNA are coloured yellow. On the basis of available crystal structures or molecular homology models, we were able to unambiguously assign density in our cryo-EM map to Rsa4, Mrt4, Nog1 and Rlp24, and suggest a likely binding site for Rlp7 ( Supplementary Table 2 ). Fitting the Mrt4 crystal structure into the Arx1 cryo-EM map To localize Mrt4 in the cryo-EM map of the Arx1 particle, we first solved the crystal structure of Mrt4 of the closely related Chaetomium thermophilum at a resolution of 1.8 Å ( Fig. 2a ; Table 1 ). Mrt4 is homologous to the ribosomal P0 protein and has been suggested to occupy its binding site on the so-called ribosomal stalk base during 60S subunit maturation [28] , [29] . Subsequently, a homology model of Saccharomyces cerevisiae Mrt4 was generated ( Supplementary Fig. 7 ) and docked into the additional density at the stalk base ( Supplementary Fig. 8 ). This revealed that the position of Mrt4 is indeed very similar to that of P0 in the mature yeast 80S ribosome [30] . Moreover, Mrt4 binds close to Nog1 (see below) and the r-protein L11 ( Fig. 2b ), with its N-terminal helix inserting between the P-stalk and rRNA helix 89. In addition, we created homology models and assigned positions for Nog1, Rlp7, Rlp24 and Rsa4. We identified Nog1 by the unique tripod-like shape of its helical N-terminal domain that blocks the premature P- and A-sites like a plug. The helix bundle forms several contacts with the 25S rRNA near helices 42, 89 and 90. The Nog1 GTPase domain binds the tip of the Sarcin–Ricin loop in close proximity to eIF6, Mrt4 and L11 ( Fig. 2c ). Our model does not include the C-terminal part of Nog1 comprising another 300 amino acids that are predicted to be unstructured ( Supplementary Table 2 ). The position of the N-terminal domain of Rlp24 was assigned to the location of L24e in the mature 60S subunit. The mostly α-helical C terminus of Rlp24 could not be assigned unambiguously. In contrast, Rlp7 appears to be part of the foot structure rather than substituting for its r-protein homologue L30 (refs 31 , 32 ). However, we found two possible albeit overlapping positions within the foot structure ( Supplementary Fig. 8 ). Finally, we observed density for Rsa4 between the rearranged 5S RNP and the stalk base. Its prominent C-terminal eight-bladed WD40 (β-propeller) domain contacts the r-proteins L18 and L11 while the N-terminal UBL (ubiquitin-like)-domain is adjacent to so far non-assigned additional densities ( Fig. 2d ). What exactly these and other unassigned extra densities represent is not clear at present. However, the amount of density corresponds well with the expected subset of additional factors biochemically identified in the early Arx1 particle. Moreover, we assume that the foot structure may additionally contain the ITS2 sequence moiety of the 5.8S rRNA with its processing factors. Figure 2: Ribosome assembly factors and their binding sites on the pre-60S subunit. ( a ) Crystal structure of Chaetomium thermophilum Mrt4 at 1.8 Å resolution. ( b ) Nog1 extends its tripod-like N-terminal domain into the distorted A- and P-sites contacting the 25S rRNA near helices 42, 89 and 90. Its GTPase domain binds to the tip of the Sarcin–Ricin loop in close proximity to eIF6, Mrt4 and L11. ( c ) Rsa4 binds between the 5S RNP and the stalk base in close proximity to L18 and L11. ( d ) Mrt4 binds to the stalk base close to Nog1 and L11. Its binding mode resembles that of P0. Protein models and crystal structures are depicted as ribbons, rRNA models (white) are depicted as density at 3.5 Å resolution, and non-interpreted density is shown in dark grey. Contact regions between ribosome assembly factors and the 25S rRNA are coloured yellow. Full size image Table 1 Data collection and refinement statistics for C. thermophilum Mrt4. Full size table Twisted topology of the 5S RNP on the pre-60S particle Apart from the presence of ribosome assembly factors, major differences between the pre-60S particle and the native 60S subunit result from rearranged rRNA itself. Most prominently, the 5S RNP was unambiguously identified in a radically different position based on the characteristic and essentially unchanged 5S rRNA fold ( Supplementary Fig. 8 ). Compared with its mature position, the 5S RNP is rotated by ~180° and the distance between the two positions of its tip spans ~130 Å ( Fig. 3 ). This premature position of the 5S RNP is accompanied by a completely rearranged central protuberance rRNA (helices 82–88) and helix 38, also known as the A-site finger. The premature and native positions of the A-site finger, respectively, enclose an angle of ~41° with the tip of the helix being repositioned by ~50 Å. In the native subunit, an important contact of the 5S RNP is established between L5 and rRNA helix 84 of the 25S rRNA. Notably, we observed the same interaction also for the premature position of the 5S RNP in the pre-60S subunit ( Fig. 4a ). This is possible due to a rotated conformation of helix 84 compared with its mature state. Together with helix 84 also the helices 82, 83 and 86 are rotated and rearranged, whereas helix 88 is already very close to its mature position ( Fig. 4b ). We detected additional conformational differences in the region of helix 69 and 71 as well as for helix 89 ( Fig. 3d ). Helix 89 was found to be much shorter than in its native state and completely relocated. Its tip occupies the binding site of L16 while its base is not yet formed. Helix 69 faces the opposite direction when compared with the native 60S subunit, and helix 71 forms a long helix sticking out of the intersubunit surface instead of adopting its reoriented and more compact mature conformation. 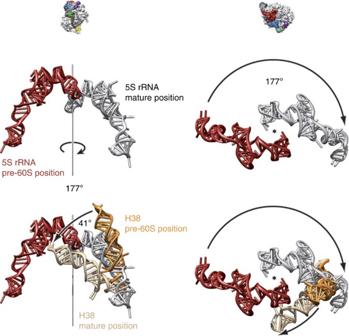Figure 3: Relation between the immature and native positions of the 5S rRNA and rRNA helix 38. The 5S rRNA and rRNA helix 38 are depicted in their respective pre-60S (red and orange) and mature (grey and light brown) positions in a side view (left) and top view (right). The location of the rotation axis for the 5S rRNA is indicated by a grey pole (left) or an asterisk (right). Figure 3: Relation between the immature and native positions of the 5S rRNA and rRNA helix 38. The 5S rRNA and rRNA helix 38 are depicted in their respective pre-60S (red and orange) and mature (grey and light brown) positions in a side view (left) and top view (right). The location of the rotation axis for the 5S rRNA is indicated by a grey pole (left) or an asterisk (right). 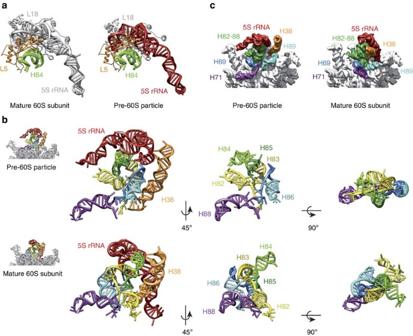Figure 4: Comparison of the 5S RNP and the central protuberance in the pre-60S particle and the mature 60S subunit. Comparison between the pre-60S and the mature state of (a) the interaction of the 5S RNP with helix 84, (b) the structure of the central protuberance rRNA and (c) the overall arrangement of the intersubunit surface rRNA. Note the distinct orientations of helices 69, 71 and 89. Full size image Figure 4: Comparison of the 5S RNP and the central protuberance in the pre-60S particle and the mature 60S subunit. Comparison between the pre-60S and the mature state of ( a ) the interaction of the 5S RNP with helix 84, ( b ) the structure of the central protuberance rRNA and ( c ) the overall arrangement of the intersubunit surface rRNA. Note the distinct orientations of helices 69, 71 and 89. Full size image Taken together, the pre-60S assembly intermediate analysed in this study displays an unforeseen but defined premature conformation of the ribosomal 25S rRNA with a markedly rearranged topology of the 5S RNP. This overall arrangement appears to be stabilized by the bound assembly factors and, thus, apparently represents an energetically favoured intermediate state along the rRNA folding/assembly pathway. The more distal biogenesis factors Rlp24 and Mrt4 apparently act as simple placeholders for their r-protein homologues, which are L24 and P0, respectively. In contrast, the more proximal factors such as Rsa4 and Nog1 contribute to the stabilization of the premature central protuberance and 5S RNP arrangement with their intricate network of interactions. The existence of such a distinct structural 60S intermediate was unpredictable and is different from recent observations in bacteria, in which the central protuberance region undergoes a transformation from a completely disordered to a near-mature state during assembly [33] . We speculate that the more distinct intermediate conformation present in eukaryotes may serve as a structural checkpoint coordinating the interaction with a specific set of biogenesis factors. When the 5S RNP rotates during subsequent maturation steps, the coupled rotation of helix 84 will also force the central protuberance helices to adopt a more native conformation and this movement will inevitably push helix 38 closer to its mature position. As such the 5S RNP may function as a wrench-like RNA chaperone before completely integrating into the native 60S subunit as a structural entity. These markedly different conformations of the rRNA can apparently provide distinct binding sites for the appropriate biogenesis factors during specific windows of the maturation process. At least one of these factors will have to provide a substantial power stroke to overcome the energy barrier between our observed immature and the native position of the 5S RNP within the maturing pre-60S particle. TAP purifications and western blotting TAP purifications of pre-60S particles (for yeast strains see Supplementary Table 3 ) were preformed in buffer containing 50 mM Tris–HCl, pH 7.5, 100 mM NaCl, 1.5 mM MgCl 2 , 5% glycerol, 0.1% NP40 and 1 mM dithiothreitol [34] . TAP-tagged proteins were affinity purified with IgG Sepharose 6 Fast Flow (GE Healthcare), followed by TEV cleavage and a second affinity step with Calmodulin Sepharose 4B (GE Healthcare). Pre-ribosomes were eluted with buffer containing 5 mM EGTA. Samples were precipitated with TCA (10%) and resuspended in SDS sample buffer. Proteins were separated on 4–12% NuPAGE polyacrylamide gels (Invitrogen). Coomassie staining and western blot analyses were preformed according to standard procedures. The following antibodies were used in this study: anti-Rpl3 1:3,000 (J.R. Warner), anti-Mex67 1:5,000 (C. Dargemont), anti-Nmd3 1:10,000 (A.W. Johnson), anti-Nop7 1:50,000 (B. Stillman), anti-Nsa3 1:2,500 (E. Tosta), anti-Rsa4 1:10,000 (M. Remacha), anti-Tif6 1:10,000 (F. Fasiolo), anti-Mrt4 1:500 and anti-P0, P1, P2 (3BH5) 1:10 (J.P. Ballesta), anti-Nug1 1:1,000 and anti-Yvh1 1:4,000 (V. Panse), anti-Arx1 1:1,000, anti-Nog1 1:5,000, anti-Nsa2 1:1,000, anti-Nug2 1:5,000, anti-Rei1 1:5,000 and anti-Rlp24 1:15,000 (M. Fromont-Racine) and secondary antibodies goat anti-rabbit (Bio-Rad #170-6515, 1:2,000) and goat anti-mouse (Bio-Rad #170-6516, 1:2,000). The split-tag purification of Arx1-TAP Flag-Rsa4 is described in more detail in the figure legend of Supplementary Fig. 5 . Cryo-EM data collection and three-dimensional reconstruction Arx1 pre-60S particles were purified using TAP-tagged Alb1, which is stably associated with Arx1 (ref. 22) [22] . The sample was applied to carbon-coated holey grids at a concentration of 2.8 OD 260 ml −1 (ref. 35 ). Micrographs were recorded under low-dose conditions (20 e − /Å 2 ) on a Titan Krios TEM (FEI Company) microscope at 200 kV in a defocus range of 1.0–3.5 μm using a TemCam F416 camera (4,096 × 4,096 pixel, TVIPS GmbH). The resulting pixel size was 1.0605 Å on the object scale. The data were processed with the SPIDER software package [36] . Images were manually inspected for good areas and power spectra. The quality of the sample as well as the grids appeared to be very high featuring optimal ice thickness and a good particle distribution for most of the micrograph images. The signature software was used to automatically pick particles from 5,686 micrographs using projections of the crystal structure of the S. cerevisiae 60S ribosomal subunit (PDB ID: 3O58) [37] as a template. Particles (263,730) were selected. To prevent model bias, the particles were initially aligned to the mature 60S ribosomal subunit. Only after the corresponding low-resolution reconstruction was found to resemble the previously published Arx1 particle [22] , this particle was then used as a reference structure to improve the yield of initially correctly aligned particles. Contaminations and non-ribosomal particles were removed by semisupervised classification using iterative multi-reference three-dimensional projection alignment [22] ( Supplementary Fig. 9 ). Out of the remaining particles a stable sub-population comprising 75,887 particles was identified and refined to 8.7 Å resolution. Model creation Starting point for the generation of the rRNA model was the crystal structure of yeast 80S ribosome (PDB ID: 3U5D) [14] . The structure was docked into the density using the UCSF chimera software (CHIMERA) [38] and divergent regions were located by visual inspection. Building blocks were cut from the structure, docked into the assigned densities and adjusted using molecular dynamics flexible fitting (MDFF) [39] . Building blocks that were not present in the template structure were taken from cryo-EM models of the yeast ribosome: ES7La (PDB ID: 3IZF), ES27L (PDB ID: 3IZD) and L1-stalk rRNA (PDB ID: 3IZF) [40] . Single-stranded linkers were manually built into the density using CHIMERA. Linkers and connections were then energy minimized by MDFF. The 5.8S rRNA remained unchanged. The r-protein model was also based on the docked crystal structure of yeast 80S ribosome (PDB ID: 3U5E). R-proteins lacking in the template structure were taken from a cryo-EM model of the yeast ribosome: L1 and L11 (PDB ID: 3IZS) [30] . For each r-protein, the presence of the corresponding density was checked and missing r-proteins were removed from the model accordingly. A loop in L6e that was not resolved in the template structure was modelled into the density using CHIMERA together with the COOT software [41] . L5 and L18 were moved into their densities as part of the 5S RNP, and L1 was shifted in order to maintain its interaction with the L1-stalk rRNA. Homology models for assembly factors (see Supplementary Table 2 ) were generated using the MPI Bioinformatics Toolkit [42] together with the MODELLER software [43] . The S. cerevisiae Mrt4 model was created using MODELLER with the C. thermophilum Mrt4 crystal structure (this study) as template after the sequences were aligned using clustalW2 (ref. 44) [44] . Densities were assigned to the models according to structural features and known interaction constraints. The models were docked into their densities using CHIMERA and then improved using MDFF. Ct Mrt4 protein expression and crystallization The C. thermophilum Mrt4-coding sequence (accession number CTHT_0025680 ) was amplified from cDNA and cloned into pET15b (Novagen) with a C-terminal 6x-His tag. Seleno-methionine (Se-Met)-labelled C. thermophilum Mrt4 was produced in E. coli BL21 (DE3) cells (Novagen) by inhibition of methionine biosynthesis and addition of Se-Met. To that end, cells were grown at 37 °C in M9 medium supplemented with 100 mg lysine, 100 mg threonine, 100 mg phenylalanine, 50 mg leucine, 50 mg isoleucine, 50 mg valine, 5 g glucose, 250 mM MgCl 2 , 1 mM CaCl 2 and 50 mg seleno- L -methionine per litre. Protein expression was induced at an OD 600 of 0.8 by the addition of 0.25 mM isopropyl-β- D -thiogalactoside. Cells were grown at 23 °C for 16 h before being harvested and stored at −80 °C. Cell pellets were resuspended in 25 ml buffer A (20 mM Hepes pH 7.5, 100 mM NaCl, 5 mM MgCl 2 , 5 mM KCl) complemented with Protease Inhibitor Mix HP (SERVA) and lysed using a M110L Microfluidizer (Microfluidics). The lysate was cleared by centrifugation (19,000 g for 30 min at 4 °C) using a JA-25.50 rotor (Beckmann). SP Sepharose beads (Sigma, cation exchange) were added to the lysate and incubated for 10 min at 4 °C. Beads were washed with 50 ml buffer A and the protein was eluted with buffer A supplemented with increasing amounts of NaCl (100 mM–1 M). Eluates from 400 to 800 mM were combined and applied to a Ni-nitrilotriacetate affinity step (buffer supplemented with 15 mM imidazole). Ni-nitrilotriacetate beads were incubated for 10 min at 4 °C and washed with four bead volumes of buffer B (20 mM Hepes pH 8.0, 200 mM NaCl, 10 mM MgCl 2 and 10 mM KCl) supplemented with 15 mM imidazole. The protein was eluted with buffer B containing 500 mM imidazole. To remove the imidazole the eluate was applied to a PD-10 column (GE Healthcare) pre-equilibrated with buffer B supplemented with 2 mM dithiothreitol. Fractions were pooled and concentrated to 20–25 mg ml −1 using an Amicon Ultracel-10K (Millipore). Crystallization screens were performed at 18 °C by sitting-drop vapour-diffusion by mixing equal volumes (0.5 μl) of protein solution (17 mg ml −1 ) and crystallization buffer. Se-Met C. thermophilum Mrt4 crystals grew in 0.1 M bicine pH 9 and 2.22 M (NH 4 ) 2 SO 4 after 2–4 days. X-ray data collection and structure determination C. thermophilum Mrt4 crystals were cryoprotected in mother liquor containing 20% (v/v) ethylene glycol and flash-cooled in liquid nitrogen. Diffraction data were measured under cryogenic conditions (100 K) on beamline ID14-4 at the European Synchrotron Radiation Facility (ESRF) in Grenoble, France. X-ray diffraction data were processed using xds and scala [45] , [46] . The initial model was obtained from a SAD Se-Met data set of Mrt4 using the AutoSol and Autobuild programs of the Phenix program suite [47] . Model building and refinement was performed with the Phenix program suite and COOT. Ramachandran statistics for the final model of C. thermophilum Mrt4 show 99.16% of residues in most favourable regions, 0.84% in additionally allowed regions and 0% in disallowed regions according to MolProbitiy [48] . Experiments were designed and the data were interpreted by C.L., M.T., I.S., E.H. and R.B. ; B.B. affinity-purified the Alb1-TAP particle and C.L. and O.B. performed the cryo-EM analysis supervised by R.B. ; M.T. preformed purifications of pre-60S particles and WB analysis and expressed and purified ct Mrt4, and I.H., G.B. and I.S. determined the crystal structure; the manuscript was written by C.L., E.H. and R.B. ; E.H. and R.B. directed the project; all authors discussed the results and commented on the manuscript. Accession codes: The coordinates of the crystal structure of ct Mrt4 have been deposited in the PDB with accession code 4NWB . The cryo-EM map has been deposited in the EMDataBank with accession code EMD-2528 and the coordinates of the model have been deposited in the PDB with accession codes 3J64 (rRNA), 3J65 (r-proteins and biogenesis factors) and 3J66 (alternative Rlp7 position). How to cite this article: Leidig, C. et al. 60S ribosome biogenesis requires rotation of the 5S ribonucleoprotein particle. Nat. Commun. 5:3491 doi: 10.1038/ncomms4491 (2014).